Tuning a Schottky barrier in a photoexcited topological insulator with transient Dirac cone electron-hole asymmetry The advent of Dirac materials has made it possible to realize two-dimensional gases of relativistic fermions with unprecedented transport properties in condensed matter. Their photoconductive control with ultrafast light pulses is opening new perspectives for the transmission of current and information. Here we show that the interplay of surface and bulk transient carrier dynamics in a photoexcited topological insulator can control an essential parameter for photoconductivity—the balance between excess electrons and holes in the Dirac cone. This can result in a strongly out of equilibrium gas of hot relativistic fermions, characterized by a surprisingly long lifetime of more than 50 ps, and a simultaneous transient shift of chemical potential by as much as 100 meV. The unique properties of this transient Dirac cone make it possible to tune with ultrafast light pulses a relativistic nanoscale Schottky barrier, in a way that is impossible with conventional optoelectronic materials. Low-energy electron bands in graphene [1] and surface states of 3D topological insulators (TIs) [2] , [3] can be described by 2D Dirac equations and are the most promising candidates for a new generation of devices based on relativistic fermions [4] . These two-dimensional dirac systems (2DDSs) represent a novel state of quantum matter characterized by revolutionary transport properties: some of these features, like the unprecedented mobility of graphene [1] or the immunity to defects and impurities of TI’s [2] , [3] , make Dirac fermions particularly interesting for ultrafast photonics and optoelectronics [5] , [6] . Their applicability to real devices requires the ability to control the lifetime and population of hot photocarriers and to manipulate the balance between excess electrons and holes in the transient regime. Several studies have already been performed to explore the response of 2DDSs to ultrafast light pulses, but none of them has focused on the effects of an asymmetric electron-hole population in the non-equilibrium Dirac cone. In the case of graphene, electron-hole symmetry has been consistently found in the photoexcited state, and it naturally stems from the direct intracone nature of the optical excitation [7] , [8] , [9] . In TIs direct optical excitation has been shown for a high-lying unoccupied surface state [10] , but for the topological surface state an excess carrier population can be instead built up in the Dirac cone via interband scattering processes involving also bulk valence and conduction states [10] , [11] , [12] , [13] , [14] , [15] . This necessarily leads to the additional problem of a strong presence of hot excess carriers in the bulk bands during the whole-transient regime following the optical excitation [11] , [12] , [13] , [14] . This is particularly disturbing in the perspective of using TIs for optoelectronic applications because one does not preserve in the photoexcited regime the essential feature of a topological insulator—the coexistence of a gapless surface state and of a bulk insulator. Here we show that these limitations can be overcome by considering an insofar neglected element: the action of the band bending on the interplay between surface and bulk carrier dynamics [16] , [17] , [18] , [19] . If correctly mastered, the band lineup can be advantageously used to control and modify the charge balance and transient population of hot Dirac fermions in a 3D TI, while keeping at the same time the subsurface space charge layer as void as possible of excess carriers. In this way, the 2DDS constitutes a strongly out of equilibrium conducting state that cannot be obtained with a conventional metal, with interesting implications for optoelectronic devices based on topological insulators. Lifetime of excited Dirac fermions We were able to unveil these effects through a series of time-resolved ARPES measurements performed on several bismuth chalcogenide TIs [20] , [21] , [22] , [23] . As representative examples, we present in Fig. 1 images obtained for selected time delays Δ t on p -type Bi 2.2 Te 3 , with a downward band bending of about 60 meV at the surface, and on Bi 2 Te 2 Se, which at 40 K is n -type [24] , [25] , [26] , [27] , [28] and presents an upward band bending of about 30 meV. For sake of comparison, in Fig. 2 we present results from a strongly n -doped Bi 2 Te 3 sample presenting flat bands at the surface. We also provide the complete time-resolved ARPES sequences for all the specimens as movies: for p -type Bi 2.2 Te 3 ( Supplementary Movie 1 ); for n -type Bi 2 Te 2 Se ( Supplementary Movie 2 ); and for strongly n -doped Bi 2 Te 3 ( Supplementary Movie 3 ). In Fig.1c we present the time evolution of the population in the k – E windows CB p *, CB n * (the bulk conduction band) and S p *, S n * (the excited Dirac cones) as defined in Fig. 1a,b for p -type Bi 2.2 Te 3 and n -type Bi 2 Te 2 Se, respectively. As discussed in previous works [11] , [14] , decay rates depend on the specific momentum-energy region: after an analysis of this dependence for our samples, detailed in the Supplementary Figure S2 , we found that this choice for the k – E windows allows us to present in Fig. 1c the essential information we need for this study. 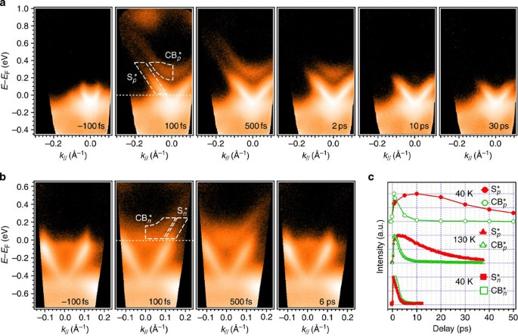Figure 1: Dirac cone ultrafast dynamics detected with time-resolved ARPES. Selected time delays are presented for (a)p-type Bi2.2Te3and (b)n-type Bi2Te2Se. The signal intensity is presented in a logarithmic colour scale. The integration regions called Sp*, Sn*, and CBp*, CBn* are indicated as dashed contour windows. (c) time evolution of Sp*, Sn*, CBp*, CBn*. Figure 1: Dirac cone ultrafast dynamics detected with time-resolved ARPES. Selected time delays are presented for ( a ) p -type Bi 2.2 Te 3 and ( b ) n -type Bi 2 Te 2 Se. The signal intensity is presented in a logarithmic colour scale. The integration regions called S p *, S n *, and CB p *, CB n * are indicated as dashed contour windows. ( c ) time evolution of S p *, S n *, CB p *, CB n *. 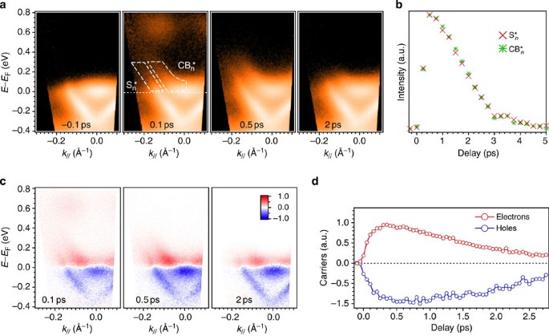Figure 2: Ultrafast dynamics of a flat band system shown for ann-type sample. (a) Time-resolved ARPES images. (b) Time evolution of the electron populations in the Dirac cone and in the conduction band: as one can see, the relaxation time for excess electrons in the Dirac cone is much faster than for thep-type sample (see alsoSupplementary Fig. S1) because in this case they are strongly coupled with the conduction band and they have access to the faster bulk carrier recombination channels. (c)k–Edistribution of excess electrons and holes; (d) time evolution of the excess electron and hole populations. As expected for a flat-band system, the electron and hole populations are very well balanced for all time delays: this becomes even more evident by comparingFig. 2(c,d) withFig. 3, where asymmetric populations are detected for excess holes and electrons, respectively. Full size image Figure 2: Ultrafast dynamics of a flat band system shown for an n -type sample. ( a ) Time-resolved ARPES images. ( b ) Time evolution of the electron populations in the Dirac cone and in the conduction band: as one can see, the relaxation time for excess electrons in the Dirac cone is much faster than for the p -type sample (see also Supplementary Fig. S1 ) because in this case they are strongly coupled with the conduction band and they have access to the faster bulk carrier recombination channels. ( c ) k – E distribution of excess electrons and holes; ( d ) time evolution of the excess electron and hole populations. As expected for a flat-band system, the electron and hole populations are very well balanced for all time delays: this becomes even more evident by comparing Fig. 2 ( c , d ) with Fig. 3 , where asymmetric populations are detected for excess holes and electrons, respectively. Full size image During the first few picoseconds an excess carrier population accumulates in the Dirac cone, as a result of different interband scattering processes that also involve bulk states, as thoroughly described in previous studies [11] , [12] . For longer delays, n -type Bi 2 Te 2 Se is almost completely relaxed after 8 ps, while in p -type Bi 2.2 Te 3 a significant population of excess hot carriers survives in the surface Dirac cone with a strikingly long lifetime of τ S ≈50 ps at T=40 K. At 130 K, this lifetime is reduced (30 ps), but it is still considerably larger than observed in previous studies on TIs [11] , [12] , [13] , [14] . By focusing our attention on the p -type specimen, it is immediately clear that after the first few picoseconds one has filled the available empty states in the Dirac cone within the gap. In Supplementary Fig. S2 we discuss this in more detail, also by comparing the results with the n -type Bi 2 Te 3 sample. It has already been observed [11] that excited surface states have a longer relaxation time when they are within the gap because they do not have access to the faster bulk recombination channels. In our case, this is very evident from the analysis of Supplementary Fig. S1 (for p -type Bi 2.2 Te 3 ) and of Fig. 2b (for n -type Bi 2 Te 3 ). Furthermore, the sequence in Fig. 1a reveals a qualitatively different process with respect to previous works on p -type Bi 2 Se 3 , where a persisting non-equilibrium population of bulk photoinduced carriers CB p * was found in the conduction band, acting as a charge reservoir for the Dirac cone states in the gap [11] , [14] . In our case, for Δ t ≳ 10 ps, the p -type Bi 2.2 Te 3 sample still presents a strong excess electron population in the surface state, while no carriers can be detected at the bottom of the conduction band. Surface band bending and transient charge asymmetry The reason for this is that a pre-existing surface band bending can strongly affect the bulk-surface interplay, and consequently the Dirac cone relaxation, by spatially separating excess electrons and holes. In our case, the inequivalent charge carrier dynamics can be extracted from the differences of the ARPES images with respect to the non-excited systems ( Fig. 3a,c ). In Fig. 3b,d we present the time evolution of the detected excess electron and hole populations. For the n -type sample, with bands slightly bent upwards, a clear excess of holes can be found in the Dirac cone for a few picoseconds. The charge asymmetry is much more pronounced for the p -type specimen. After 500 fs, the hole population starts decreasing in the surface layers (with 6.3 eV photons our ARPES probing depth is about 2–3 nm (ref. 29 )) while excess electrons maintain a strong presence as they are actually trapped in the surface states (see also Fig. 3a ). This is due to the surface band bending, which induces a flow of the excess majority carriers (holes) towards the bulk, while the excess minority carriers (electrons) remain confined at the surface. This charge disequilibrium at the surface explains the unusually long relaxation time for Bi 2.2 Te 3 (excess electrons find no holes to recombine with), as well as its temperature dependence (the bulk mobility of the carriers is lower at 40 K than at 130 K due to impurity scattering). The corresponding transient surface photovoltage [30] , [31] was measured for the various time delays ( Supplementary Fig. S3 ) and found to be negligibly small (≈10 meV) for the laser fluences used in this study. 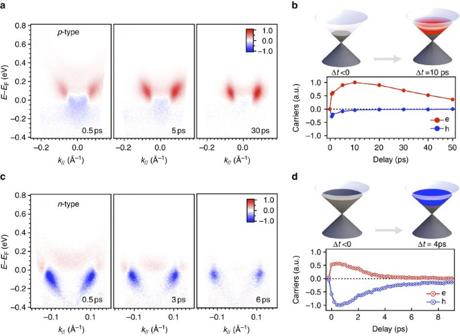Figure 3: Charge asymmetry of transient excess carriers. Excess electrons (red) and holes (blue) are detected from the difference of time-resolved ARPES images taken after and before photoexcitation. We present them in (a) forp-type Bi2.2Te3and in (c) forn-type Bi2Te2Se. In (b,d) we present the time evolution of the detected excess carriers (electrons, e and holes, h): a transient accumulation of holes is seen for then-type specimen and a much more pronounced asymmetry related to a strong and long-lived accumulation of hot electrons in the Dirac cone for thep-type sample. Figure 3: Charge asymmetry of transient excess carriers. Excess electrons (red) and holes (blue) are detected from the difference of time-resolved ARPES images taken after and before photoexcitation. We present them in ( a ) for p -type Bi 2.2 Te 3 and in ( c ) for n -type Bi 2 Te 2 Se. In ( b , d ) we present the time evolution of the detected excess carriers (electrons, e and holes, h): a transient accumulation of holes is seen for the n -type specimen and a much more pronounced asymmetry related to a strong and long-lived accumulation of hot electrons in the Dirac cone for the p -type sample. Full size image Electron-hole asymmetry as a carrier recombination bottleneck The lack of holes in the surface and subsurface region acts as the effective bottleneck for the recombination of excess Dirac electrons, which present an unusually long lifetime for the basic reason that there are not enough positive charge carriers to recombine with. If the bands are instead flat, the distribution of excess bulk electrons and holes is essentially always balanced (in time t and in space z ), and the recombination of excess Dirac carriers will be mainly limited by intrinsic factors, like the electron-phonon scattering rate. This is indeed the case for the flat-band n -type Bi 2 Te 3 sample presented in Fig. 2 , as well as for a prototype system where no surface-bulk interplay is present, namely non-equilibrium Dirac cones in graphene [7] , [8] . In the case of 3D TIs, various time-resolved ARPES studies have examined how the weak electron-phonon coupling determines the slow relaxation of the surface states: in particular the sibling compound Bi 2 Se 3 has already been extensively explored [11] , [13] , [14] , [15] for different temperatures and for pump fluences ranging from 0.025 to 0.25 mJ cm −2 , with relaxation rates for the Dirac cone excess population between 5 and 10 ps. Here we are confronted with a markedly different time scale for the Dirac cone relaxation (of the order of 50 ps or more, and strongly dependent on the sample temperature), which is due to a different underlying physical process, namely the transient macroscopic charge carrier separation. This is unambiguously confirmed by the fact that the relaxation time was found to increase even more when the bands were more bent. We were able to perform this test by letting a cleaved surface exposed to the residual gases of our ultrahigh vacuum system: consistent with previous studies [32] , [33] , after 24 h we observed an increase of surface band bending increased, and we found that the Dirac cone relaxation rate as well (see Fig. 4 ). This is possible thanks to the well-known robustness of the surface of topological insulators and indicates possible practical pathways to actively control this effect. 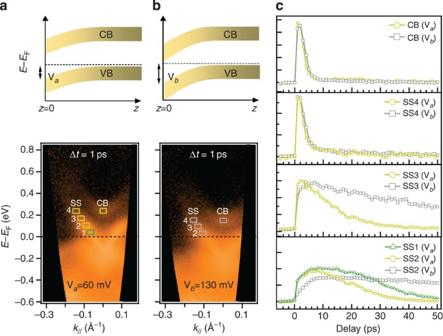Figure 4: Effect of band bending on the recombination rate forp-type Bi2.2Te3. Decay rates for photoexcited p-Bi2.2Te3at T=40 K in the case of (a) a Va=60 mV band bending and (b) of a Vb=130 mV band bending (b). The pump-probe ARPES images correspond to a time delay of 1 ps. In (c) the decay rates for equivalent energy windows are compared. The energy windows for the surface state SS have been chosen so that SS4 has the same binding energy as the bottom of the conduction band CB. As it can be clearly seen, equivalent windows for the two surfaces show a much longer relaxation time for surface (b), where the band bending is more pronounced. In particular, SS2 for the case (b) has a lifetime ≥100 ps (there is of course no equivalent in (b) of window SS1 because, due to the increased band bending, in (b) SS1 becomes part of the filled electronic states). Figure 4: Effect of band bending on the recombination rate for p -type Bi 2.2 Te 3 . Decay rates for photoexcited p-Bi 2.2 Te 3 at T=40 K in the case of ( a ) a V a =60 mV band bending and ( b ) of a V b =130 mV band bending ( b ). The pump-probe ARPES images correspond to a time delay of 1 ps. In ( c ) the decay rates for equivalent energy windows are compared. The energy windows for the surface state SS have been chosen so that SS4 has the same binding energy as the bottom of the conduction band CB. As it can be clearly seen, equivalent windows for the two surfaces show a much longer relaxation time for surface ( b ), where the band bending is more pronounced. In particular, SS2 for the case ( b ) has a lifetime ≥100 ps (there is of course no equivalent in ( b ) of window SS1 because, due to the increased band bending, in ( b ) SS1 becomes part of the filled electronic states). Full size image Transient topological insulator state In Fig. 5 we illustrate the consequences of the spatial separation of photoexcited negative and positive carriers for the case where they are more pronounced and long lasting, that is, for p -type Bi 2.2 Te 3 (specular arguments may be applied to the case of n -type Bi 2 Te 2 Se). The photoexcited excess electrons, confined to the subsurface region, fill the surface Dirac cone over few picoseconds, and, after 10 ps, there are no visible electrons in the conduction band. There are also no excess holes in the subsurface valence band because they have drifted deeper into the bulk ( z ≳ L D , where L D is the Debye length of the system); furthermore, for (0≤ z ≲ L D ) the Fermi level is really within the band gap. Consequently, within the space charge layer (that is, the subsurface region corresponding to 0≤ z ≲ L D ) a situation is created where there is a strong excess population of electrons concentrated in the conducting surface states while no excess carriers are present in the bulk bands: therefore, the space charge layer preserves also in the transient regime this main distinctive feature of TIs. If one gates the system on a time window starting 10 ps after the pump pulse, this portion of the specimen can consequently be regarded as a genuine transient topological insulator, whose extension in space ( L D ≈20 nm) and in time (Δ t ≈50 ps) can be interesting for ultrafast optoelectronic applications. 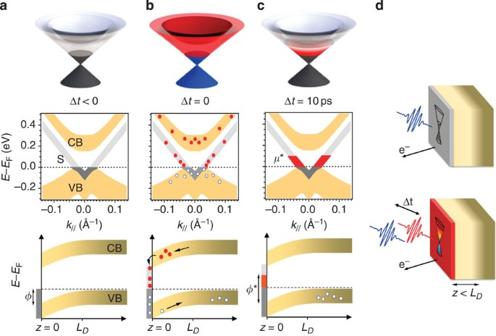Figure 5: Transient topological insulator state and non-equilibrium surface 2D metallic layer in a nanoscale Schottky barrier. We compare Bi2.2Te3(a) in its ground state, (b) right after photoexcitation and (c) in its photoexcited state for a delay Δt=10 ps after optical pumping. For each case, the top panel represents a pictorial view of the Dirac cone with excess electrons (red) and holes (blue); the mid panel shows the schematic structure of the bands in reciprocal space and their filling at the surface (z=0); and the bottom panel the corresponding band lineup in real space along the normal to the surfacez. In (d) we present a schematic view of the experimental configuration: when the sample is in its ground state (top), ARPES probes the rest valueφof the barrier between the chemical potentialμand the top of the valence band; when the sample is photoexcited with a pump pulse, time-resolved ARPES probes the evolution of the transient topological insulator state versus time delay Δt(bottom): the difference of the Schottky barrier heightφ*−φis only due to the strongly out of equilibrium 2DDS. Figure 5: Transient topological insulator state and non-equilibrium surface 2D metallic layer in a nanoscale Schottky barrier. We compare Bi 2.2 Te 3 ( a ) in its ground state, ( b ) right after photoexcitation and ( c ) in its photoexcited state for a delay Δ t =10 ps after optical pumping. For each case, the top panel represents a pictorial view of the Dirac cone with excess electrons (red) and holes (blue); the mid panel shows the schematic structure of the bands in reciprocal space and their filling at the surface ( z =0); and the bottom panel the corresponding band lineup in real space along the normal to the surface z . In ( d ) we present a schematic view of the experimental configuration: when the sample is in its ground state (top), ARPES probes the rest value φ of the barrier between the chemical potential μ and the top of the valence band; when the sample is photoexcited with a pump pulse, time-resolved ARPES probes the evolution of the transient topological insulator state versus time delay Δ t (bottom): the difference of the Schottky barrier height φ *− φ is only due to the strongly out of equilibrium 2DDS. Full size image Phototuning of a relativistic Schottky barrier In order to appreciate the character of this transient state, we can consider it as a nanometer scale metal-semiconductor junction between the metallic 2DDS and the subsurface space charge layer. In its ground state, the chemical potentials μ of the 2DDS and of the substrate are in equilibrium, and the energy difference between the top of the valence band and μ can be regarded as the height φ of the Schottky barrier ( Fig. 5 ). The transient filling of the Dirac cone after photoexcitation can be regarded as a shift of a chemical potential defined only for the surface 2DDS, μ *. In the transient topological insulator state (Δ t ≳ 10 ps), the substrate bands are virtually the same as in the ground state, but the barrier height of the Schottky barrier has changed by about 0.1 eV, that is, more than half the gap of Bi 2.2 Te 3 . Even more remarkably, this large change is only due to the shift of μ * in the 2DDS, which in this transient regime is not in equilibrium with the substrate. It should be emphasized that for junctions between a semiconductor and a normal metal the Schottky barrier height can be changed in many ways, but these methods always involve changing the lineup of the semiconductor bands, while the metal side is unaffected [34] . In the current case, it is instead the metallic side that is strongly perturbed: this is a consequence of the unique properties of the 2DDSs at the surface of TIs, namely the fact that they simultaneously present a metallic nature and an exceptionally long relaxation time for their photoexcited state. Analysis of the non-equilibrium Dirac cone A detailed analysis of the energy distribution curves (EDCs) gives a more complete description of the evolution of this strongly out of equilibrium Dirac cone. In Fig. 6a we consider momentum-selected EDCs taken along the surface bands of p -type Bi 2.2 Te 3 at T=130 K, and we present in the contour plot the difference of the photoexcited Dirac cone with respect to its equilibrium state. In Fig. 6b we present the EDCs in logarithmic scale for two limiting cases, Δ t <0 (non-excited state) and 0.5 ps (strongly out of equilibrium state). The momentum-selected EDC for Δ t <0 can be well fitted with a Fermi-Dirac distribution, with T e =130 K, convoluted with our experimental resolution (80 meV). The spectrum for Δ t =0.5 ps presents a non-zero signal level at high kinetic energies, a background due to incoming scattered electrons. To model the EDC, we describe this background with a constant energy distribution D 2 * for E ≥ E F , plus a Fermi-Dirac distribution with temperature T e and chemical potential μ * to describe the rest of the excess population D 1 *. This model makes the assumption that an electronic temperature T e can be defined for a subset of the overall electron population, neglecting D 2 *, and it provides a good fit for the spectra at all delays (as it can be seen for selected time delays in Fig. 6b ). The parameters extracted from the fit are plotted in Fig. 6c and indicate that a real electronic thermalization develops only when D 2 *=0 and when μ * reaches its maximum value (for Δ t = τ t , with τ t =4 ps at T=130 K, Fig. 6d ). Strictly speaking, when D 2 *≠0 parameters like μ * and T e are physically ill-defined, and we report them in Fig. 6c with different symbols for the sake of clarity. This distinction is particularly clear here because the band filling (Δ t ≤ τ t ) and its quasi-adiabatic relaxation (Δ t ≥ τ t ) takes place on well distinct time scales [35] . Hence, for the transient topological insulator state (Δ t ≥10 ps) a quasi-equilibrium chemical potential for the Dirac cone can be rigorously defined; this corresponds to the μ * introduced in Fig.5 . 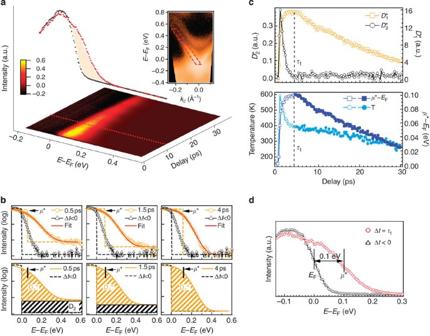Figure 6: Transient electronic temperature and chemical potential of non-equilibrium Dirac fermions. (a) Contour plot of the energy-time distribution of transient hot carriers in the surface Dirac cone of p-type Bi2.2Te3at 130 K. The two spectra above the contour plot are two representative momentum-selected EDCs extracted from the integration area indicated in the inset, for Δt=10 ps and Δt<0 ps, respectively; the excess electron population is represented by the shaded area between them, and it corresponds to the color scale in the 2D plot. (b) Top panels: momentum-selected EDC’s at Δt=0.5, 1.5 and 4 ps with relative fitting curves, and their difference with respect to the EDC taken at Δt<0 ps; bottom panels: visualisation for the various time delays ofD1* andD2*, parameters used to fit the transient electronic states with a Fermi-Dirac distribution as explained in the text. (c) Time evolution of the fitting parameters. (d) Comparison of the momentum-selected EDCs for the Dirac cone at equilibrium and for Δt=τt. Figure 6: Transient electronic temperature and chemical potential of non-equilibrium Dirac fermions. ( a ) Contour plot of the energy-time distribution of transient hot carriers in the surface Dirac cone of p-type Bi 2.2 Te 3 at 130 K. The two spectra above the contour plot are two representative momentum-selected EDCs extracted from the integration area indicated in the inset, for Δ t =10 ps and Δ t <0 ps, respectively; the excess electron population is represented by the shaded area between them, and it corresponds to the color scale in the 2D plot. ( b ) Top panels: momentum-selected EDC’s at Δ t =0.5, 1.5 and 4 ps with relative fitting curves, and their difference with respect to the EDC taken at Δ t <0 ps; bottom panels: visualisation for the various time delays of D 1 * and D 2 *, parameters used to fit the transient electronic states with a Fermi-Dirac distribution as explained in the text. ( c ) Time evolution of the fitting parameters. ( d ) Comparison of the momentum-selected EDCs for the Dirac cone at equilibrium and for Δ t = τ t . Full size image From the fundamental point of view, this state represents a model case of universal relevance for a non-equilibrium fermion distribution and shows that electron-hole asymmetry in the subsurface carrier population can be a more stringent factor in the relaxation of a hot 2DDS than intrinsic processes like electron-phonon scattering. It should be emphasized that only the combination of the unique intrinsic properties of the 2DDS and of its interplay with the semiconductor substrate make it possible to drive a metallic state in such a markedly out of equilibrium state. The key for achieving this condition is that the intrinsically slow recombination time for the surface states is long enough to give subsurface excess majority carriers the time to drift into the bulk. For example, for the case of the p -type specimen discussed in this paper, the time necessary to create a strong electron-hole asymmetry in the subsurface region and in the surface bands (few picoseconds, see Figs 3a and 5b ) is faster than the intrinsic Dirac cone relaxation, primarily determined by electron–phonon scattering. At this point (approximately at t = τ t ) the still very high number of excess electrons in the Dirac cone are left with an insufficiently small number of holes to recombine with: as the total electrical charge must be conserved during the recombination process, the asymmetry between electrons and holes becomes the most stringent bottleneck for their recombination, which is consequently further slowed down to a considerably longer time scale (of the order of 50 ps). The necessity of this simultaneous combination of different factors explains why such a long-lived, strong shift of the chemical potential has never been observed for a metallic system (neither for a metallic film at a junction with a semiconductor nor for a 3D metal). From the point of view of possible technological applications, it is well known that a precise control of the chemical potential position is a key issue and one of the main challenges towards the realization of materials with genuine TI properties [2] , [3] , that is, systems where the chemical potential is in the middle of the bulk band gap, the Dirac cone is partially occupied and there are no excess carriers in the bulk bands. The transient state described in this paper does present all these properties, and it demonstrates that manipulating TIs with ultrafast light pulses can provide alternative and powerful pathways for the control of their unique transport properties. In particular, we have observed that for an electron (or hole) travelling along the z direction, the 2DDS at the surface of a 3D TI represents a Schottky barrier. As we have discussed, an advantageous time window exists in the transient regime such that the space charge layer region 0≤ z ≲ L D can be found in virtually the same state as before photoexcitation, while the 2DDS presents a photoshifted chemical potential: this system represents a potentially interesting photoexcited TI, where the Schottky barrier height can be transiently tuned with ultrafast light pulses. This can be used for instance in a new type of transiently tuneable Schottky diodes based on Dirac fermions, by selectively acting with nanoscale electrical contacts only on the space charge layer region. The possibility we described of maintaining a genuine TI also in the photoexcited state is of relevance for any photoconductive application of this kind of 2DDS, especially if one considers that the thickness of the space charge layer region (around 20 nm) is comparable to the penetration length of optical photons in the material. In general, our findings are of interest for any kind of applications where one wants to use light to transfer electrons from the semiconducting substrate to the surface 2DDS, or conversely if one wants to prevent this transfer. In conclusion, our results indicate a general approach to effectively photoinduce a strongly out of equilibrium state by acting on the charge balance in the Dirac cone of TIs. This photoexcited 2DDS simultaneously presents a metallic nature and an extremely long recombination time; it may for instance be used in a nanometer scale Schottky photodiode because the 2DDS is simultaneously atomically thin and strongly, topologically decoupled from the substrate. All these properties cannot be found in a conventional metal and indicate many interesting perspectives for the ultrafast photoconductive control of 2DDSs. In the case of graphene, a strong photoinduced electron-hole asymmetry could be produced with the use of high energy photons, involving indirect scattering with higher energy bands: this could be very interesting in combination with the realisation of graphene-based metal-semiconductor contacts [36] . For TIs, additional opportunities are related to the possibility of actively exploiting the helical spin texture of the Dirac fermions in optospintronics. The photon energy and the electric field related to band bending, along with the relative position of the Fermi level and of the Dirac point, are the main factors determining the properties of the excited Dirac cone. As all these factors can be tailored at will using adjustable parameters, they appear to be essential tools for future devices based on the photoconductive control of Dirac fermions. Transport measurements The high quality single crystals used for these experiments were thoroughly characterized before the time-resolved ARPES experiments. The growth of the Bi 2 Te 2 Se crystals employed in this study had been described elsewhere [24] , as has their basic electronic characterization [24] , [25] . The Bi 2.2 Te 3 and Bi 2 Te 3 crystals were grown by following the Bridgman method, and their transport properties have been determined by measuring their longitudinal and transverse Hall resistivities. Six gold contacts were evaporated on the samples in a standard geometry. From these measurements, the resistivity and conductance tensors can be fully extracted after symmetrization (antisymmetrization) of the longitudinal (transverse) resistivities with respect to the magnetic field, which was applied perpendicular to the layers. In addition, thermopower experiments were also performed on both materials as a function of temperature. The analysis of the Hall coefficients ( Supplementary Fig. S4 ) and Seebeck coefficients ( Supplementary Fig. S5 ) allowed us to conclude that the Bi 2 Te 3 specimen was strongly n -doped, with a bulk carrier density n ≈10 21 cm −3 . The Bi 2.2 Te 3 was instead p -doped, with a bulk hole carrier density n h ≈9 × 10 18 cm −3 . Time-resolved ARPES measurements The band lineup was precisely determined by comparing the bulk carrier concentration extracted from transport measurements with the band position observed with surface sensitive ARPES on clean, freshly cleaved specimens. The time-resolved ARPES measurements were performed on the FemtoARPES setup, in experimental conditions similar to our previous work [12] . The laser source was operated at 0.25 MHz repetition rate, pumping the specimens with 1.57 eV pulses (35 fs, 0.1 mJ cm −2 ) and probing them with the 4th harmonic at 6.3 eV (ref. 37 ), with an overall time resolution of 65 fs and an energy resolution of 80 meV. The data presented here were taken along ΓK direction, but we found no substantial differences for measurements performed along other directions in k -space on several cleaved surfaces, obtaining consistently similar results for the dynamics of the excited states. How to cite this article: Hajlaoui, M. et al. Tuning a Schottky barrier in a photoexcited topological insulator with transient Dirac cone electron-hole asymmetry. Nat. Commun. 5:3003 doi: 10.1038/ncomms4003 (2014).